A real-time study of the benefits of co-solvents in polymer solar cell processing The photoactive layer of organic solar cells consists of a nanoscale blend of electron-donating and electron-accepting organic semiconductors. Controlling the degree of phase separation between these components is crucial to reach efficient solar cells. In solution-processed polymer–fullerene solar cells, small amounts of co-solvents are commonly used to avoid the formation of undesired large fullerene domains that reduce performance. There is an ongoing discussion about the origin of this effect. To clarify the role of co-solvents, we combine three optical measurements to investigate layer thickness, phase separation and polymer aggregation in real time during solvent evaporation under realistic processing conditions. Without co-solvent, large fullerene-rich domains form via liquid–liquid phase separation at ~20 vol% solid content. Under such supersaturated conditions, co-solvents induce polymer aggregation below 20 vol% solids and prevent the formation of large domains. This rationalizes the formation of intimately mixed films that give high-efficient solar cells for the materials studied. Focussed research efforts on organic semiconductors have pushed the certified efficiency of single junction organic solar cells to over 10% (ref. 1 ). To become a viable technology, research is now focussing on stability and lifetime [2] , [3] as well as all-solution, roll-to-roll compatible production routes [4] , [5] and the use of environmental friendly solvents [6] , [7] . It is well known that the morphology of organic solar cells is crucial to achieve high efficiencies. New materials require new solvents and new processing conditions to be identified that provide an optimized morphology. This may involve thermal annealing, solvent vapour annealing or the use of co-solvents [8] , [9] . In fact, the use of co-solvents has become ubiquitous but it remains a skill rather than being based on a deep understanding of the dynamical processes that occur during solution processing of the organic layer. This work aims to investigate the formation of the photoactive layer in real time during spin coating and elucidate the role of co-solvents. Processing polymer solar cells with a co-solvent involves spin coating of a four-component mixture: the polymer donor and fullerene acceptor are dissolved in a main solvent together with a small amount (1–10 vol%) of co-solvent. Empirically, it has been established that successful co-solvents have a higher boiling point than the main solvent and provide a higher solubility for the fullerene derivative than for the polymer [10] . For some polymer–fullerene combinations, it was shown that the effect of a co-solvent is to increase domain sizes [11] , which is most commonly attributed to polymer aggregation in solution [12] , [13] . Contrastingly, for other combinations, the function of the co-solvent is to decrease domain sizes. In several polymer–fullerene blends, large (>100 nm) droplet-shaped fullerene-rich domains are formed when the film is cast without co-solvent. It has been shown that these large fullerene domains can originate from liquid–liquid phase separation during solvent evaporation [14] , [15] . When the same blend is processed with a suitable co-solvent, the large droplet-shaped domains are not found and a much more intimately mixed morphology is formed that provides increased photovoltaic performance [15] . Among the materials that show such behaviour there are several that provide very high power conversion efficiencies (PCEs) in solar cells. A prominent example is PTB7 that provides a well mixed blend and PCE=9.2% when processed with co-solvents [16] , but forms large (>100 nm) fullerene-rich domains and correspondingly low PCEs when processed from a single solvent [17] , [18] , [19] . Other examples that give similar behaviour are PDPPTPT (PCE=7.4%) (refs 20 , 21 ), PDTG-TPD (PCE=7.4%) (refs 22 , 23 ), PBnDT-FTAZ (PCE=7.0%) (ref. 24 ), PBDTTPD (PCE=8.3%) (ref. 25 ) and P(iI-DTS) (PCE=4%) (ref. 26 ). In Supplementary Fig. 1 , we show the structures of these polymers to show their widely different chemical composition. The origin of the decrease of domain size when using a co-solvent has often been attributed to polymer aggregation, either in the casting solution [27] , [28] or during solvent evaporation [18] , [29] . It has also been ascribed to a reduction of fullerene aggregation in the casting solution [30] . The lack of consensus regarding the role of co-solvents arises, in part, from the inability to study the morphology formation during realistic device processing conditions. In situ studies that are performed during solvent evaporation can shed light on these processes. Liu et al . [18] , [29] studied the drying of a blade-coated and drop-cast films in which a co-solvent decreases domain sizes. However, during spin coating, the complex morphologies develop in a few seconds, which is much faster than the drying of blade-coated or drop-cast films, which takes 1,000 s or more. The dynamics of solvent evaporation and phase separation govern the final structure. In situ studies have been performed on timescales corresponding to realistic processing conditions for practical applications [31] , [32] , [33] , [34] . However, in none of these systems co-solvents are necessary to decrease domain sizes. In the following, we monitor layer thickness, polymer aggregation and large-scale phase separation during spin coating. We show for the first time that without the co-solvent, polymer aggregation occurs after large-scale liquid–liquid phase separation. Using a co-solvent, the aggregation of the polymer occurs at higher solvent content. Enough co-solvent has to be added to ensure that the onset of polymer aggregation occurs before large-scale phase separation can occur. The effect of co-solvents on efficiency and morphology For our study, we use an alternating diketopyrrolopyrrole-quinquethiophene copolymer donor (PDPP5T) in combination with phenyl-C 71 -butyric acid methyl ester ([70]PCBM) as fullerene acceptor ( Fig. 1a ). DPP-based copolymers have emerged as versatile small band gap semiconductors and provide PCEs up to 8% in combination with [70]PCBM [35] . Processing PDDP5T and [70]PCBM (1:2 w/w) into an efficient photoactive layer requires the use of co-solvents [36] . For the PDPP5T:[70]PCBM blend, we studied the effect of co-solvent on device performance for two commonly used co-solvents: ortho-dichlorobenzene (oDCB) and diiodooctane (DIO). 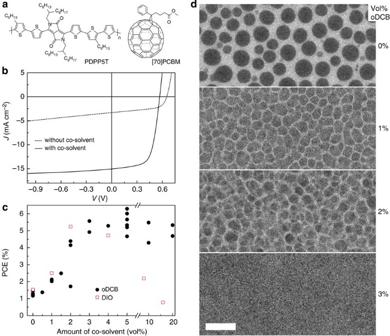Figure 1: The influence of co-solvent on performance and morphology. (a) Chemical structure of PDPP5T and [70]PCBM. (b)J–Vcurves under simulated solar illumination of PDPP5T:[70]PCBM (1:2 w/w) solar cells processed from chloroform without and with 3 vol% oDCB. (c) The effect of the concentration of co-solvent on the PCE for oDCB and DIO. (d) Bright-field TEM images of PDPP5T:[70]PCBM (1:2 w/w) films spin coated from chloroform with the indicated amount of oDCB as co-solvent. Scale bar, 600 nm. Figure 1b shows the distinct difference in the current density–voltage ( J – V ) characteristics for layers processed from chloroform without and with 3 vol% oDCB as co-solvent. Figure 1c shows the PCE as a function of the used concentration (vol%) of co-solvent (oDCB or DIO). Without co-solvent, the PCE of this material combination is less than 2%. The PCE reaches a maximum above 5% for oDCB concentrations above 3 vol% and remains high when the concentration is increased up to 20 vol%. For DIO, the maximum PCE is found for 2 vol% and it decreases again rapidly above 4 vol%. Figure 1: The influence of co-solvent on performance and morphology. ( a ) Chemical structure of PDPP5T and [70]PCBM. ( b ) J–V curves under simulated solar illumination of PDPP5T:[70]PCBM (1:2 w/w) solar cells processed from chloroform without and with 3 vol% oDCB. ( c ) The effect of the concentration of co-solvent on the PCE for oDCB and DIO. ( d ) Bright-field TEM images of PDPP5T:[70]PCBM (1:2 w/w) films spin coated from chloroform with the indicated amount of oDCB as co-solvent. Scale bar, 600 nm. Full size image The strong effect of the co-solvent on the PCE relates to the morphology as evidenced by transmission electron microscopy (TEM, Fig. 1d ). Using no co-solvent, large (that is, >100 nm) [70]PCBM-rich domains are formed in a polymer-rich matrix. This morphology originates from the liquid–liquid phase separation during drying: due to solvent evaporation, the mixture enters the spinodal region of the ternary phase diagram [15] , in which rapid amplification of thermal fluctuations in composition results in [70]PCBM-rich droplets in a polymer-rich solution, that persist until the film is dry. The large domains that form are detrimental for the PCE because the electrons generated in the mixed, polymer-rich, matrix cannot be collected efficiently [15] , [37] . The domain size decreases for 1 and 2 vol% oDCB, although larger features remain visible. At 3 or more vol% oDCB these larger structures are absent and the morphology appears to be a finely blended bulk heterojunction, wherein most photogenerated excitons can be dissociated and contribute to current generation. A similar effect of co-solvent on morphology is seen when DIO is used ( Supplementary Fig. 2 ); however, only 2 vol% of DIO is enough to decrease the domain size to an optimum. Spin coating dynamics studied by real-time measurements To understand the formation of these blend morphologies, it is important to investigate the dynamics of the relevant processes during spin coating. We use three optical techniques that provide real-time information on film thickness, liquid–liquid phase separation and polymer aggregation during spin coating. For film thickness, we monitor the intensity of specular reflected laser light with a photodiode during spin coating. Owing to the decreasing layer thickness, conditions for constructive and destructive interference occur remittently ( Fig. 2a ). After determining the final (dried) layer thickness, a peak-counting method is used to back-calculate the wet layer thickness during drying [38] . Owing to solvent evaporation, at some point the mixture may enter a spinodal region and become unstable such that liquid–liquid phase separation occurs. This causes a refractive index contrast between the fullerene-rich droplets and the polymer-rich solution. Consequently, the droplets will scatter light ( Fig. 2b ) and the onset of liquid–liquid phase separation can be detected by the onset of light scattering, which is measured simultaneously with the film thickness by a second photodiode positioned at an off-specular angle. 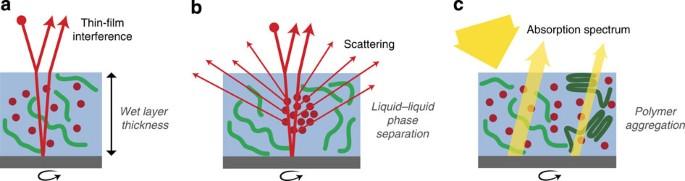Figure 2: Real-time optical analysis of film formation. (a) The interference of incident laser light is monitored to measure the solvent layer thickness during drying as function of time. (b) Scattered laser light monitors the onset of liquid–liquid phase separation. (c) A change in the diffuse reflection of white light detected the change in the absorption spectrum that accompanies aggregation of polymer chains in solution. Figure 2: Real-time optical analysis of film formation. ( a ) The interference of incident laser light is monitored to measure the solvent layer thickness during drying as function of time. ( b ) Scattered laser light monitors the onset of liquid–liquid phase separation. ( c ) A change in the diffuse reflection of white light detected the change in the absorption spectrum that accompanies aggregation of polymer chains in solution. Full size image The results of the two combined interference and scattering measurements are shown in Fig. 3 . The top panel of Fig. 3 shows the film thickness as a function of time, reconstructed from the interference signal. When spin coated from pure chloroform, the PDPP5T:[70]PCBM layer is dry within 0.8 s. The thickness curve clearly shows two phases: first, thinning is mainly caused by radial spreading of material. After that, the decrease in thickness becomes linear with time, which indicates that thinning is solely caused by solvent evaporation. The onset of a scattering signal is readily detected in the solvent evaporation phase (indicated by the dashed dark blue line in the bottom panel) and indicates the onset of liquid–liquid phase separation. Using the reconstructed thickness data and the dry layer thickness, the solvent concentration at the onset of phase separation is calculated to be 83±3 vol% for this example. 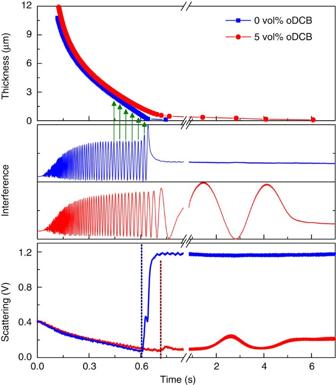Figure 3: Detecting liquid–liquid phase separation with time. Film thickness, normalized interference and light scattering of PDPP5T:[70]PCBM in solvent mixtures is monitored during spin coating at 2,000 r.p.m. The solvent is chloroform (blue squares) and chloroform with 5 vol% oDCB (red circles). Green arrows schematically indicate the thickness reconstruction from the measured interference signal. The dashed lines indicate the onset of scattering. Figure 3: Detecting liquid–liquid phase separation with time. Film thickness, normalized interference and light scattering of PDPP5T:[70]PCBM in solvent mixtures is monitored during spin coating at 2,000 r.p.m. The solvent is chloroform (blue squares) and chloroform with 5 vol% oDCB (red circles). Green arrows schematically indicate the thickness reconstruction from the measured interference signal. The dashed lines indicate the onset of scattering. Full size image Using 5 vol% oDCB in chloroform, the drying time increases from 0.8 to 6 s (note the axis break in Fig. 3 ). After the initial flow phase, there is a stage where mainly chloroform evaporates until ~0.7 s. In the final 5 s mainly oDCB evaporates. This implies that during these last 5 s the oDCB concentration is much larger than 5 vol%. In part, this explains why such a seemingly low amount of co-solvent can have such a dramatic effect. With oDCB, there is no strong scattering signal, but there is a small step indicated by the dark red dashed line. As will be shown later, this is probably due to small inhomogeneities caused by polymer aggregation. An interference effect can also be seen in the light scattering signal. This is explained by the fact that interference effects cause light intensity fluctuations in the wet layer. Using DIO as a co-solvent, a somewhat different interference pattern is found. When measurements are done for a characteristic spin-coating time (~60 s), only a chloroform-drying regime is observed. A 7,000-s spin-coating experiment reveals that DIO evaporates on much longer timescales (see Supplementary Fig. 3 ). For a DIO concentration of 4 vol%, drying continues for 56 min while spinning continuously at 2,000 r.p.m. Such long spin coating is not commonly used and hence DIO-processed layers typically remain wet until a high-vacuum step is employed. For normal spin-coating times (1–2 min), it is likely that the solids:DIO ratio in the chloroform-dried film is the same as their initial ratio. Monitoring polymer aggregation during spin coating Apart from liquid–liquid phase separation, aggregation of the polymer chains occurs during spin coating and drying of the films. To detect this aggregation, the substrates were modified as shown in Supplementary Fig. 4 . A white paint layer is applied on the backside of a glass substrate. On the topside of the glass substrate a titanium oxide (TiO 2 ) layer is added to provide refractive index contrast to enable simultaneous interference experiments. On top of the TiO 2 a PEDOT:PSS layer is used to mimic the substrate properties used in regular solar cells. The white paint is illuminated through the wet layer and the substrate by focussed light from a halogen lamp. The white paint scatters this light, which is then transmitted for a second time through the whole layer stack ( Fig. 2c ). The off-specular scattered light is collected by a fibre optic cable. The fibre optic cable is connected to a spectrometer to acquire in situ absorption spectra. 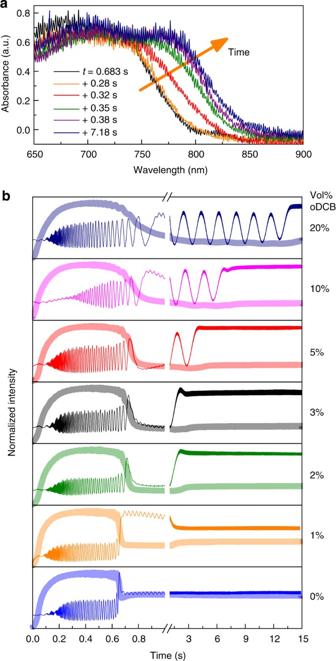Figure 4: Detecting polymer aggregation with time. (a) Evolution of the absorption spectrum during spin coating of a PDPP5T:[70]PCBM film from chloroform with 3 vol% oDCB. (b) Laser interference (thin lines) and transmission of 780–820 nm light (thick semi-transparent lines) of PDPP5T:[70]PCBM films during spin coating from chloroform with different concentrations oDCB. Figure 4a shows the changes in the absorption for a PDPP5T:[70]PCBM (1:2 w/w) blend spin coated from chloroform with 3 vol% oDCB. Directly after starting the spin coating, a decrease of absorption in the flow phase was observed (see Supplementary Movie 1 , until t =0.68 s), due to material that is radially ejected from the substrate. In the subsequent solvent evaporation phase ( Fig. 4a ), a red shift of the optical absorption can be seen ( t =0.96–1.06 s). It is well known that the aggregation of π-conjugated polymers causes a red shift in the absorption spectrum [39] , and experiments as shown in Fig. 4a reveal when this process occurs. Figure 4: Detecting polymer aggregation with time. ( a ) Evolution of the absorption spectrum during spin coating of a PDPP5T:[70]PCBM film from chloroform with 3 vol% oDCB. ( b ) Laser interference (thin lines) and transmission of 780–820 nm light (thick semi-transparent lines) of PDPP5T:[70]PCBM films during spin coating from chloroform with different concentrations oDCB. Full size image To measure polymer aggregation simultaneously with layer thickness via interference experiments, a band-pass filtered photodiode is used which only collects light between 780–820 nm. The red shift in absorption can then be detected as a decrease in transmitted light intensity. The results are shown in Fig. 4b for different concentrations of oDCB, and for different concentrations of DIO in Supplementary Fig. 5 . The decrease in transmission always occurs during the transition from the chloroform-drying to the oDCB-drying regime. The oDCB-drying regime takes much longer with increasing amounts of co-solvent and shows more interference peaks. Hence, for higher oDCB concentrations, polymer aggregation occurs in thicker wet layers with a higher total solvent content. In addition, aggregation takes longer and there is a larger change in transmission for higher oDCB concentrations, indicating that the extent of aggregation increases. As shown in Supplementary Fig. 6 , this shifts the absorption onset in the dry films and decreases the open-circuit voltage, in agreement with results obtained by Kim et al . [40] The solvent content at the onset of phase separation The total solvent concentrations where polymer aggregation starts, as calculated from these experiments for oDCB and DIO in chloroform, are shown in Fig. 5a,b as blue circles; the pink stars represent the onset of the scattering signal. Without the co-solvent, the onset of scattering occurs before the decrease in transmission. This implies that in pure chloroform liquid–liquid phase separation precedes polymer aggregation. Raising the amount of co-solvent to ~2–4 vol% increases the solvent content at which the transmission change occurs, while the onset of scattering still occurs at approximately the same solvent content. The onsets of liquid–liquid phase separation and polymer aggregation occur at approximately the same solvent concentration, and thus time, for co-solvent concentrations of 2 vol%. For even higher co-solvent contents, the change in transmission and scattering signal occur at the same time, indicating that polymer aggregation is the cause of the (small) scattering signals. 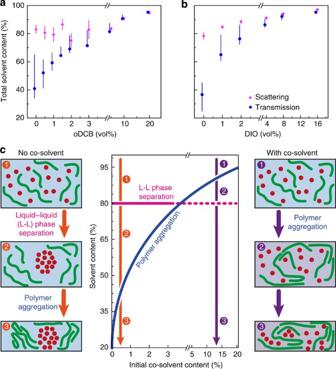Figure 5: Which is first: phase separation or polymer aggregation? (a) Total solvent content (concentration in vol%) at the onset of scattering (pink stars) and at the change in transmission (blue circles at 50% change) versus concentration of oDCB in the initial chloroform solution (error bars for scattering arise from the time-uncertainty in the scattering onset; thickness uncertainty from back-calculating the interference signals is not included. The transmission error bars indicate 20–80% transmission change). (b) Same for DIO instead of oDCB. (c) Schematic phase diagram revealing the role of co-solvent in inducing polymer aggregation at higher solvent contents which, in turn, prevents large-scale liquid–liquid phase separation during drying and results in optimized morphologies. Figure 5: Which is first: phase separation or polymer aggregation? ( a ) Total solvent content (concentration in vol%) at the onset of scattering (pink stars) and at the change in transmission (blue circles at 50% change) versus concentration of oDCB in the initial chloroform solution (error bars for scattering arise from the time-uncertainty in the scattering onset; thickness uncertainty from back-calculating the interference signals is not included. The transmission error bars indicate 20–80% transmission change). ( b ) Same for DIO instead of oDCB. ( c ) Schematic phase diagram revealing the role of co-solvent in inducing polymer aggregation at higher solvent contents which, in turn, prevents large-scale liquid–liquid phase separation during drying and results in optimized morphologies. Full size image Phase separation in other polymer–fullerene blends To test the generality of these results, we studied two more polymers. The two polymers consist of a DPP unit alternating with a sequence of thiophene–phenyl–thiophene (TPT) rings along the chain, but differ with respect to the length of the sides chains. The shorter 2-hexyldecyl (HD) side chains of PDPPTPT-HD result in a reduced solubility compared to PDPPTPT-DT with longer 2-decyltetradecyl (DT) side chains. For PDPPTPT-HD:[70]PCBM, PCEs over 7% have been obtained [20] , [35] . For both derivatives, the solvent content at the onset of scattering and at the change in transmission were measured ( Supplementary Fig. 7 ) for solutions in pure chloroform and in chloroform with an optimized amount of co-solvent. Liquid–liquid demixing precedes polymer aggregation in films that are processed from solutions of PDPPTPT-HD or PDPPTPT-DT with [70]PCBM in pure chloroform. However, when using a co-solvent, the onset of polymer aggregation occurs before liquid–liquid phase separation can occur. These results are fully consistent with those obtained for PDPP5T and [70]PCBM. Role of the co-solvents Our interpretation of this data is clarified in Fig. 5c . The orange arrow indicates the order of events when no co-solvent is used: (1) when spin coating is started, the chloroform concentration decreases due to evaporation; (2) at ~80 vol% total solvent content liquid–liquid phase separation occurs; (3) at ~50 vol% total solvent content the polymer aggregates. The domain size is determined in step (2) by the fullerene droplets which are formed by liquid–liquid phase separation. When co-solvents are used, the purple arrow indicates the order of events: (1) the total solvent content decreases mainly due to chloroform evaporation, thus the solvent quality for the polymer decreases; (2) at ~80–95 vol% total solvent content the polymer starts aggregating; (3) the polymer has aggregated before liquid–liquid phase separation has occurred, and no large domains are formed. For both co-solvents, the onset of aggregation and scattering seem to start overlapping around 2% co-solvent content ( Fig. 5a,b ). Because the high molecular weight fraction of PDPP5T is essentially insoluble in oDCB and in DIO, it is not surprising that the onsets of aggregation are similar for the two co-solvents. The 2% co-solvent contents is also the minimal amount of co-solvent that needs to be added to make high-performing solar cells with small domain sizes ( Fig. 1 ). In these experiments, large-scale phase separation does not occur if the onset of polymer aggregation occurs simultaneously with or before the unstable spinodal regime in the phase diagram is entered. These results qualitatively agree with in situ X-ray analyses of a blade-coated PTB7:[70]PCBM film and a drop-cast PDPP4T:[70]PCBM sample using a co-solvent as reported by Liu et al . [18] , [29] For both systems, polymer aggregation occurs when the fullerene is still dissolved. Liu et al . propose that the formation of polymer networks prevents large-scale domain formation. Effect of polymer preaggregation Combined, these observations seem to indicate that polymer aggregation prevents liquid–liquid phase separation. To test this hypothesis, solar cells were made using a solution in pure chloroform. PDPP5T and [70]PCBM were dissolved by stirring for 60 min at 90 °C. This solution was allowed to preaggregate for 6 days during which it remains very fluid (not gelated) and without visible precipitation. Atomic force microscopy (AFM) of photoactive layers of solar cells spin coated from this preaggregated solution ( Fig. 6a ) clearly show that liquid–liquid phase separation has occurred. The external quantum efficiency (EQE, Fig. 6c ) shows a pronounced red-shifted response, caused by the preaggregated polymer. The absorption spectra recorded during drying of these films ( Fig. 6d ) evidence that the polymer had already aggregated in the casting solution. The onset of absorption is similar for the preaggregates in solution and film. The same solution was then restirred for 20 min at 90 °C to redissolve the aggregates and cooled to room temperature for 10 min. 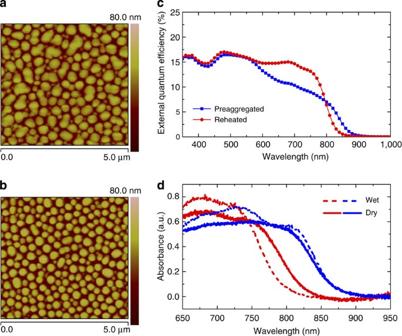Figure 6: Aggregation alone does not prevent liquid–liquid demixing. (a) AFM height image of the photoactive layer of a solar cell made from a PDPP5T:[70]PCBM solution in pure chloroform which had been left to preaggregate for 6 days. (b) AFM height image of a the photoactive layer of solar cell made from the same solution as inathat had been restirred at 90 °C for 20 min and left to cool down for 10 min to room temperature before spin coating. (c) EQE measurements of the solar cells inaandbreveal that the solar cell from the preaggregated solution has a more pronounced red-shifted response and a slightly lower photocurrent compared to the solar cell from the reheated solution. (d)In situabsorption spectra showing wet and dry film absorption spectra for both solar cells ina(preaggregated) andb(reheated). The measurements were vertically shifted such that the absorbance at 925 nm is set to zero. The thickness of the active layers of both solar cells was 100 nm. Figure 6d shows that this removes the preaggregates from the solution and therefore results in liquid–liquid phase separation ( Fig. 6b ) when spin coating a film. Both the EQE ( Fig. 6c ) and the changes in the spectrum recorded in situ ( Fig. 6d ) show that the polymer aggregates formed by preaggregation have a more pronounced red-shifted absorption onset than the aggregates formed in situ by spin coating the reheated solution. Hence, the nature of the aggregates might be different. These experiments demonstrate that aggregation by itself is not enough to prevent liquid–liquid phase separation. Figure 6: Aggregation alone does not prevent liquid–liquid demixing. ( a ) AFM height image of the photoactive layer of a solar cell made from a PDPP5T:[70]PCBM solution in pure chloroform which had been left to preaggregate for 6 days. ( b ) AFM height image of a the photoactive layer of solar cell made from the same solution as in a that had been restirred at 90 °C for 20 min and left to cool down for 10 min to room temperature before spin coating. ( c ) EQE measurements of the solar cells in a and b reveal that the solar cell from the preaggregated solution has a more pronounced red-shifted response and a slightly lower photocurrent compared to the solar cell from the reheated solution. ( d ) In situ absorption spectra showing wet and dry film absorption spectra for both solar cells in a (preaggregated) and b (reheated). The measurements were vertically shifted such that the absorbance at 925 nm is set to zero. The thickness of the active layers of both solar cells was 100 nm. Full size image To prevent the liquid–liquid phase separation, the co-solvent induced aggregation must occur under supersaturated conditions at 5 to 20 vol% solid content in a mixture that is enriched in the co-solvent, which is a poor solvent for PDPP5T. We hypothesize that under these supersaturated conditions, the polymer gelates by forming a fibrillar network, which rapidly increases the viscosity and thus prevents large-scale morphology development, or that the polymer precipitates which prevents liquid–liquid phase separation by altered interactions between the components as a consequence of the enrichment of the solution with co-solvent and reduced concentration of dissolved polymer. In summary, we have shown that the combination of three relatively simple in situ real-time measurements can elucidate the complex processes that occur during the rapid drying of four-component solar cells blends. For two popular co-solvents and three different polymer–fullerene combinations, we have shown that the co-solvent causes the onset of polymer aggregation to occur before liquid–liquid phase separation. When this aggregation occurs under supersaturated conditions, the formation of large [70]PCBM-rich domains is prevented. Because many polymer:fullerene blends exhibit very similar morphological changes when using co-solvents [16] , [17] , [18] , [19] , [20] , [21] , [22] , [23] , [24] , [25] , [26] , it is of interest to study if the proposed mechanism has wider applicability and to what extend other effects contribute. The in situ methods outlined in our study can be used for this purpose and can likely be transferred to the in-line monitoring of drying processes in roll-to-roll deposition. Understanding the mechanisms underlying the morphology formation will provide a more straightforward optimization of solar cell processing conditions. This is a necessary development considering the challenges that remain for organic solar cells to become a viable technology. Substrate preparation Three different substrates were used: (1) Solar cells are made on prepatterned indium-tin-oxide substrates (Naranjo Substrates); (2) combined interference and scattering was performed on silicon substrates (Si-Mat, 525 μm thickness with 200 nm SiO 2 layer); (3) interference and absorption and transmission measurements were done on glass slides. All substrates were thoroughly cleaned by sonication in acetone, scrubbing and sonication in a sodium dodecyl sulfate solution (99%, Acros), rinsing with deionized water and finally sonication in 2-propanol. Then, on substrate type (3), a titanium oxide layer was prepared using a sol-gel method. Acetylacetone (50 μl, 99+%, Acros) and titanium(IV) isopropoxide (145 μl, 97%, Aldrich) were added to 2-proponol (1.0 ml), spin coated at 2,000 r.p.m. and baked for 30 min at 400 °C. Later, a latex-based white paint was spin coated on the backside of the slide at 800 r.p.m. Before application of the photoactive layer, all substrates were treated with ultraviolet-ozone and covered with a 40-nm thick poly(ethylenedioxythiophene):poly(styrene sulfonate) (PEDOT:PSS, Heraeus Clevios PVP Al 4083) layer. Solar cell fabrication For the active layer PDPP5T [36] was mixed with [70]PCBM (Solenne BV, 90–95%) and dissolved in chloroform with various amounts of co-solvents by overnight stirring at 65 °C. DIO (98%) and oDCB (99%) were supplied Sigma-Aldrich. The mass loading was 6 mg ml −01 for PDPP5T and 12 mg ml −1 for [70]PCBM. Spin coating was done at 2,000 r.p.m. in air at room temperature. At room temperature, [70]PCBM is well soluble in chloroform (61 mg ml −1 ) (ref. 41 ), in oDCB (203 mg ml −1 ) (ref. 41 ) and in DIO (63 mg ml −1 ) (ref. 42 ). PDPP5T is only soluble in chloroform. In oDCB, only a low molecular weight fraction of PDPP5T can dissolve ( Supplementary Fig. 8 ) and it is essentially insoluble in DIO. For solar cells, a back electrode was evaporated consisting of LiF (1 nm) and Al (100 nm). Solar cell characterization Current density–voltage ( J–V ) characteristics were measured by sweeping the voltage from −2 to +2 V using a Keithley 2400 sourcemeter. A tungsten halogen lamp was used in conjunction with a Hoya LB120 daylight filter to simulate the solar spectrum. The total light intensity was checked with a calibrated Si photodiode to be ~100 mW cm −2 . EQE was measured with a chopper-modulated 50 W Philips focusline tungsten halogen lamp in combination with an Oriel Cornerstone 130 monochromator. The modulated signal was amplified by a current preamplifier (Stanford Research System Model SR570) and measured by a lock-in amplifier (Stanford research Systems SR830). The measurements were converted to EQE by using a calibrated silicon reference cell. Real-time measurements For interference and scattering experiments, a 632.8-nm HeNe laser (5 mW, Melles-Griot) was used. The laser beam was spread to a spot of ~3 mm radius using a biconvex lens, which removes disturbances caused by the rotating sample by averaging over a larger area. A diffuser was used to collect all specular reflected light and to filter out a slight wobble in the spinning disk. An Si photodiode (Thor Labs SM1PD1A) collected the light behind the diffuser. A current preamplifier (Stanford Research System Model SR570) operating in high-bandwidth mode amplified the short-circuit current of the photodiode. A photodiode (Hamamatsu S2281) collected off-specular scattered light under a ~45° angle, which was amplified by a second current preamplifier. A Keithley 2636 A sourcemeter simultaneously measured both amplified signals as a voltage. For the thickness calculation, Wolfram Mathematica 9.0 was used to automatically select peaks and valleys in the interference signals, which was always manually checked. Using the final dry layer thickness (measured with a Veeco Dektak 150 profilometer), the thickness was backwards reconstructed from the interference signal by repetitive addition of λ /(4 n cos θ ) (amounting to ~100 nm per peak-valley distance). Here θ is the angle of incidence of the laser on the substrate and λ is the wavelength of the laser. The approximate volume fractions of all components were used to estimate the refractive index n . For absorption and transmission experiments, a light from halogen lamp was focussed on approximately the same area as the laser light. To avoid heating, a relatively low light intensity was used. A fibre optic cable collected the light that was transmitted through the layer stack, scattered by the white paint and again transmitted through the whole stack. A spectrometer (Avantes Avaspec-2048 × 14) was used in store-to-RAM mode. Raw counts are transformed to an absorption spectrum using , where I m indicates the wavelength-dependent amount of counts. The subscript dark is a dark reference and blank is a reference measurement on the substrate before spin coating the active layer. For photodiode-based transmission measurements, a band-pass filter (centred at 800 nm, FWHM 40 nm) was used in front of a Si photodiode (Thor Labs SM1PD1A). This signal was measured in the same way as the scattering signal. Morphology characterization and thickness measurement For TEM, PDPP5T:[70]PCBM films were floated from the PEDOT-covered indium-tin-oxide substrates on 200 square mesh copper grids. TEM was performed with a Tecnai G2 Sphera (FEI) operating at 200 kV. Tapping-mode AFM was performed using a Veeco MultiMode AFM with Nanosensor PPP-NCHR-50 tips. How to cite this article : van Franeker, J. J. et al . A real-time study of the benefits of co-solvents in polymer solar cell processing. Nat. Commun. 6:6229 doi: 10.1038/ncomms7229 (2015).